Abstract rule neurons in the endbrain support intelligent behaviour in corvid songbirds Despite the lack of a layered neocortex and fundamental differences in endbrain organization in birds compared with mammals, intelligent species evolved from both vertebrate classes. Among birds, corvids show exceptional cognitive flexibility. Here we explore the neuronal foundation of corvid cognition by recording single-unit activity from an association area known as the nidopallium caudolaterale (NCL) while carrion crows make flexible rule-guided decisions, a hallmark of executive control functions. The most prevalent activity in NCL represents the behavioural rules, while abstracting over sample images and sensory modalities of the rule cues. Rule coding is weaker in error trials, thus predicting the crows’ behavioural decisions. This suggests that the abstraction of general principles may be an important function of the NCL, mirroring the function of primate prefrontal cortex. These findings emphasize that intelligence in vertebrates does not necessarily rely on a neocortex but can be realized in endbrain circuitries that developed independently via convergent evolution. The last common ancestor of birds and mammals lived some 300 million years ago [1] , at a time when the six-layered neocortex, which gives rise to sophisticated cognition in primates, had not yet developed from the pallium of the endbrain [2] , [3] . Since then, many features of the pallial endbrain (telencephalon) have evolved independently and distinctly in the different sauropsid (reptiles and birds) and mammalian lineages, respectively. However, despite fundamental differences in endbrain organization, highly intelligent species evolved from both vertebrate classes through convergent evolution. Corvids (jays, jackdaws, crows and ravens), the largest songbirds, are probably the most successful family of birds that populate almost every ecological niche. The cognitive capabilities of different corvid species are impressive and rival primates [4] . For instance, corvids manufacture and use tools [5] , take the presence of conspecifics into account [6] , [7] , exhibit episodic-like memory [4] , flexibly provide for future needs [8] , master elaborate tests of object permanence [9] , [10] and—like other songbirds—exhibit vocal learning [3] . Corvids seem to extract general principles to guide behaviour quite swiftly. In laboratory tests of executive control, corvids readily transferred rules underlying matching or oddity discrimination to new sets of stimuli [11] , while pigeons seem to require a substantially larger set of training examples to show reliable transfer of general concepts [11] , [12] , [13] . The emergence of sophisticated executive control functions in corvids has important implications for our understanding of intelligence. This is because birds lack a prefrontal cortex (PFC) that in primates operates at the apex of the cortical hierarchy and orchestrates perception, thought and action in accordance with internal goals [14] , [15] . Therefore, understanding the differences and similarities of neuronal processing in two fundamentally differently organized endbrains of distantly related species will help to reveal the general computational principles underlying cognitive behaviour and executive control functions. The origins and evolution of the avian endbrain and the mammalian neocortex, where complex cognitive functions are centred, have been studied intensively. Both the pallial components of birds and the neocortex of mammals originate from the telencephalic pallium and are thus homologous as a whole [2] , [3] —that is they evolved from the same structure in a common ancestor. In pigeons, the nidopallium caudolaterale (NCL) of the endbrain has been identified as a key cognitive brain component, similar to the PFC in mammals [16] . Lesion and recording studies in pigeons demonstrated the NCL’s importance for cognition (for example, working memory, reversal learning and reward prediction) [17] , [18] , [19] , [20] , [21] . Moreover, the two areas share important properties such as dense innervation by dopaminergic fibres and connectivity patterns with multiple sensory input, limbic and motor output regions [16] . However, the pattern of thalamic connections [22] as well as developmental gene expression patterns [23] , [24] and differences in macroarchitectures in birds versus mammals suggest that NCL and PFC are not homologous—that is, they independently evolved from different parts of the pallium [25] , [26] . Therefore, the avian NCL is considered to be a functional analogue of the mammalian PFC [14] , a structure with similar function but different evolutionary origin. Despite corvids’ remarkable behavioural flexibility, the neural substrate and mechanisms of cognitive control in corvids are unexplored. Anatomical investigations show that the neural substrates to support higher cognitive abilities are disproportionately increased in the corvid family. The relative brain weight measures are unusually high in corvids [27] , [28] , and endbrain association areas such as the nidopallium are proportionally larger in corvids compared with other songbirds [29] . We therefore investigated the neuronal processing underlying task switching based on rules, a classical executive function task used in monkeys [30] , [31] , [32] , [33] , [34] , in behaving carrion crows. We report that the most prevalent single-cell activity represents behavioural rules in an abstract manner and can predict the crows’ behavioural decisions. This suggests that the abstraction of general rules and principles might be an important function of the NCL, mirroring the function of primate PFC. Such data will help to decipher the general principles and evolutionary constraints for the design of highly cognitive vertebrate brains. Crows flexibly applied abstract rules To test the neuronal foundation of executive control functions in corvids, we trained two carrion crows ( Corvus corone corone ) to switch flexibly between two general rules in a delayed match/nonmatch-to-sample task. The ‘match’ rule required crows to peck at a test object that was identical to a preceding sample object, whereas the ‘nonmatch’ rule required a peck to the test object that was different (nonidentical) from the sample object ( Fig. 1 ). A cue presented in the delay period between the sample and the test epochs indicated the appropriate rule for the current trial. To distinguish neural activity related to the rule from activity related to sensory properties of the cue, each rule was instructed by two different cues from different sensory modalities (auditory and visual), while opposite rules were indicated by two cues from the same modality [30] . The ‘match’ rule was indicated by either a blue circle or a auditory upward sweep. In contrast, the ‘nonmatch’ rule was cued either by a red circle or by a white-noise sound. Only one rule cue was presented in each trial, and all four rule cues were presented pseudorandomly interleaved within a session. 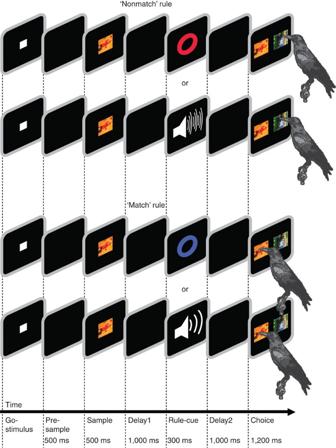Figure 1: Behavioural protocol. The birds initiated a trial by moving their heads in front of the screen during presentation of the go-stimulus. A sample stimulus was presented for 500 ms, followed by a 1,000 ms delay. A rule cue (either auditory or visual) instructed the bird about the current rule (‘match/nonmatch’), followed by a second 1,000 ms delay. In the choice period, crows pecked either at the image identical to or different from the sample, according to the previously indicated rule, to receive a reward. All relevant task parameters were balanced. Figure 1: Behavioural protocol. The birds initiated a trial by moving their heads in front of the screen during presentation of the go-stimulus. A sample stimulus was presented for 500 ms, followed by a 1,000 ms delay. A rule cue (either auditory or visual) instructed the bird about the current rule (‘match/nonmatch’), followed by a second 1,000 ms delay. In the choice period, crows pecked either at the image identical to or different from the sample, according to the previously indicated rule, to receive a reward. All relevant task parameters were balanced. Full size image Both crows performed well above chance and reliably switched between the tasks (90.8 and 91.1% correct performance; all performance levels P <0.001, Binomial test, number of trial repetitions n given in Fig. 2a ). To test whether the crows were following abstract rules and not stimulus-specific response associations, we presented a transfer session with trial-unique sample and nonmatch pictures, which the crows had never seen before. Performance in this transfer test was indistinguishable from regular performance ( P >0.05 χ 2 test, number of trial repetitions n given in Fig. 2b ). Moreover, performance on the first trials for each of the 16 sample-rule cue combinations in a session was high (90.4 and 93.2% correct for the two birds) and not statistically different from performance on the respective last trials (93.8 and 93.6% correct; both P >0.05, Wilcoxon-signed rank test, n =16), indicating that the birds did not acquire fixed sample-rule cue-specific response associations within a daily recording session, even if the same four sample pictures were used throughout one session. This demonstrates that the crows indeed grasped the ‘match’/’nonmatch’ concept in an abstract way and could flexibly apply it to arbitrary stimuli. 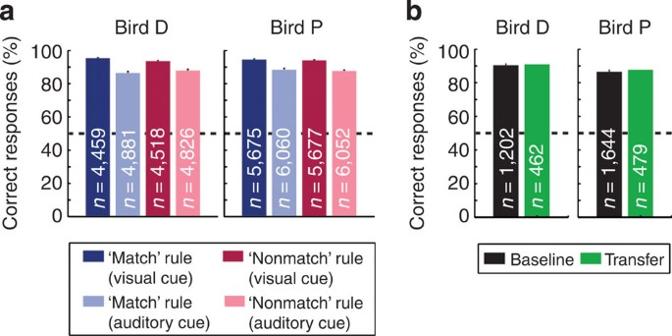Figure 2: Behavioural performance. (a) Behavioural performance (percent correct) for bird P and bird D for the two different rules and the four different rule cues. Error bars show s.e.m. over all recording sessions. Dashed lines indicate chance level. (b) Behavioural performance in a transfer session consisting of 420 unique trials, compared against baseline performance measured in three sessions for each bird. Error bars show s.e.m., dashed lines indicate chance level. Figure 2: Behavioural performance. ( a ) Behavioural performance (percent correct) for bird P and bird D for the two different rules and the four different rule cues. Error bars show s.e.m. over all recording sessions. Dashed lines indicate chance level. ( b ) Behavioural performance in a transfer session consisting of 420 unique trials, compared against baseline performance measured in three sessions for each bird. Error bars show s.e.m., dashed lines indicate chance level. Full size image Identification of the corvid NCL based on dopaminergic input As the NCL has only been investigated in pigeons so far, we identified the carrion crow’s NCL for physiological recordings. We applied immunohistochemical tyrosine hydroxylase (TH) staining of brain sections to demarcate the NCL in the corvid brain based on its dense dopaminergic innervation [35] , [36] ( Fig. 3 ). 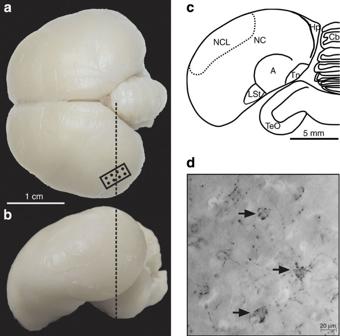Figure 3: The brain of the carrion crow. (a) Dorsal and (b) lateral view of the crow’s brain. Vertical dashed line indicates section level A5.00 shown inc. The dots inarepresent penetration sites of the eight electrodes (2 × 4 grid). (c) Coronal section (A5.00 level indicated by dashed vertical line ina) through the brain of a carrion crow illustrating the borders of the NCL in the caudal telencephalon based on immunohistochemistry for tyrosine hydroxylase.A, Arcopallium;Cb, Cerebellum;Hp, Hippocampal formation;LSt, striatum laterale;NC, Nidopallium caudale;NCL, Nidopallium caudolaterale;Tn, Nucleus taeniae amygdalae;TeO, Tectum opticum. (d) Magnified brain section (coronal plane) from the NCL. Tyrosine hydroxylase-immunoreactive fibres surround perikarya to form ‘baskets’ (arrows). ‘Baskets’ were numerous in the neuropil of the NCL. Figure 3c shows the borders of the stained area, which contained characteristic ‘basket’ structures that are characterized by TH-positive fibres coiled up like baskets around unlabelled perikarya ( Fig. 3d ). Electrodes were implanted above the NCL in the two trained crows ( Fig. 3a,b ). The location of the electrodes was histologically verified to lie in the NCL in a different crow, which was implanted with the same stereotaxic coordinates. Figure 3: The brain of the carrion crow. ( a ) Dorsal and ( b ) lateral view of the crow’s brain. Vertical dashed line indicates section level A5.00 shown in c . The dots in a represent penetration sites of the eight electrodes (2 × 4 grid). ( c ) Coronal section (A5.00 level indicated by dashed vertical line in a ) through the brain of a carrion crow illustrating the borders of the NCL in the caudal telencephalon based on immunohistochemistry for tyrosine hydroxylase. A , Arcopallium; Cb , Cerebellum; Hp , Hippocampal formation; LSt , striatum laterale; NC , Nidopallium caudale; NCL , Nidopallium caudolaterale; Tn , Nucleus taeniae amygdalae; TeO , Tectum opticum. ( d ) Magnified brain section (coronal plane) from the NCL. Tyrosine hydroxylase-immunoreactive fibres surround perikarya to form ‘baskets’ ( arrows ). ‘Baskets’ were numerous in the neuropil of the NCL. Full size image Population activity in NCL reflected the behavioural rules We recorded single-cell activity of 336 neurons in the NCL of the endbrain of the two trained carrion crows ( Fig. 4a–c ). The location of recorded units within the 2 × 4 electrode grid (depicted in Fig. 3a ) is shown in Fig. 4d for bird D and in Fig. 4e for bird P. We first applied population analyses based on the entire sample of recorded neurons. To quantify the time course of task variables (behavioural rule, cue modality and their interaction) encoded by the population of all recorded neurons, we calculated the percent variance explained by each factor ( ω 2 ) ( N =336; Fig. 5a ). In the cue and early Delay2 period, the activity was dominated by sensory properties of the rule cue (cue modality); however, information about the behavioural rule emerged as the strongest factor influencing the firing rates of all neurons towards the end of the Delay2 period. In addition, we performed a sliding decoding analysis using a k-Nearest-Neighbor classifier [37] (see Methods, Fig. 5b ) to determine whether the discharge rates present in the neuronal population could successfully predict the different task parameters. The k-Nearest-Neighbor algorithm classifies each trial based on the class of its closest neighbouring trials in the feature space of the firing rates of all recorded neurons ( Fig. 5b ). Therefore, it does not make assumptions about the underlying distribution of firing rates. Decoding of the cue modality was perfect immediately after the onset of the rule cue but declined rapidly with time during the trial. In contrast, information about the rule emerged slower after rule-cue onset and remained almost perfect throughout the Delay2 phase ( Fig. 5c ). This demonstrates that the neuronal population as a whole successfully carried the rule information through the Delay2 until a behavioural choice was required. 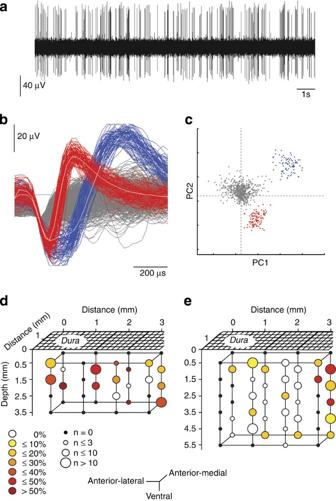Figure 4: Single-unit recordings and location of recording sites in NCL. (a) Example of a 15-s recording trace from the NCL of a behaving carrion crow, recorded with a 2-MΩ electrode. (b) Action potential waveforms (red and blue, respectively) of two isolated NCL neurons. (c) The same waveforms as inbshown in the two-dimensional principal component space (PC1 versus PC2) used to sort single units. Two single-unit waveforms cluster together (redandblue) and are separated from each other and the noise distribution (grey). (d) NCL recording sites of bird D in the 2 × 4 grid of electrodes at different depths. The size of the dots represents the number of recorded units at each location, the colour represents the percentage of rule-selective neurons recorded at each location. (e) NCL recording sites of bird P, same layout as ind. Figure 4: Single-unit recordings and location of recording sites in NCL. ( a ) Example of a 15-s recording trace from the NCL of a behaving carrion crow, recorded with a 2-MΩ electrode. ( b ) Action potential waveforms (red and blue, respectively) of two isolated NCL neurons. ( c ) The same waveforms as in b shown in the two-dimensional principal component space (PC1 versus PC2) used to sort single units. Two single-unit waveforms cluster together ( red and blue ) and are separated from each other and the noise distribution ( grey ). ( d ) NCL recording sites of bird D in the 2 × 4 grid of electrodes at different depths. The size of the dots represents the number of recorded units at each location, the colour represents the percentage of rule-selective neurons recorded at each location. ( e ) NCL recording sites of bird P, same layout as in d . 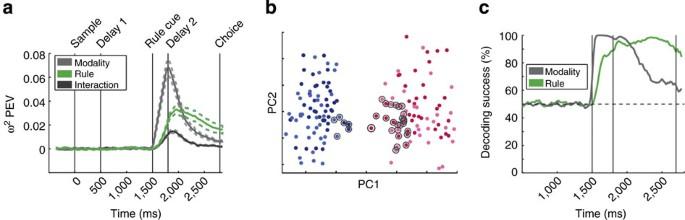Figure 5: Rule selectivity of neurons in the NCL. (a) Percent-explained variance (PEV) by the factors ‘cue modality’ and ‘behavioural rule’ for the entire population of recorded neurons, calculated in a 300 ms-sliding window using theω2statistic. At the beginning of the Delay2, there was a strong sensory influence by the cue modality. At the end of the Delay2 period, the abstract behavioural rule was the strongest variable accounting for the variance in firing rates. Vertical lines mark transitions between task periods, dashed lines show s.e.m. (b) k-Nearest-Neighbor classification: the feature space, spanned by the firing rates of all neurons in a late window. To reduce dimensionality, only the first two principal components (PC1 and PC2) are shown. Each trial is assigned the same label as the majority vote of its k-nearest neighbours in the training set. Neighbours are those trials with the smallest Euclidean distance in the feature space. Blue dots represent trials where the ‘match’ rule was shown, pink dots represent trials where the ‘nonmatch’ rule was shown. An example test trial is marked with a black circle, its nearest neighbours are marked with grey circles. Since the majority of the neighbours belong to the pink class (‘nonmatch’ rule), the test trial would be classified (correctly) as belonging to the pink class. (c) Performance of a k-Nearest-Neighbor classifier predicting the behavioural rule in each trial from the firing rates of all recorded neurons (green). Performance of a second k-Nearest-Neighbor classifier predicting the cue modality in each trial from the firing rates of all recorded neurons (grey). Dashed line indicates chance level. Vertical lines mark the beginning of the rule-cue period, end of the rule-cue period and end of the Delay2 period. Full size image Figure 5: Rule selectivity of neurons in the NCL. ( a ) Percent-explained variance (PEV) by the factors ‘cue modality’ and ‘behavioural rule’ for the entire population of recorded neurons, calculated in a 300 ms-sliding window using the ω 2 statistic. At the beginning of the Delay2, there was a strong sensory influence by the cue modality. At the end of the Delay2 period, the abstract behavioural rule was the strongest variable accounting for the variance in firing rates. Vertical lines mark transitions between task periods, dashed lines show s.e.m. ( b ) k-Nearest-Neighbor classification: the feature space, spanned by the firing rates of all neurons in a late window. To reduce dimensionality, only the first two principal components (PC1 and PC2) are shown. Each trial is assigned the same label as the majority vote of its k-nearest neighbours in the training set. Neighbours are those trials with the smallest Euclidean distance in the feature space. Blue dots represent trials where the ‘match’ rule was shown, pink dots represent trials where the ‘nonmatch’ rule was shown. An example test trial is marked with a black circle, its nearest neighbours are marked with grey circles. Since the majority of the neighbours belong to the pink class (‘nonmatch’ rule), the test trial would be classified (correctly) as belonging to the pink class. ( c ) Performance of a k-Nearest-Neighbor classifier predicting the behavioural rule in each trial from the firing rates of all recorded neurons ( green ). Performance of a second k-Nearest-Neighbor classifier predicting the cue modality in each trial from the firing rates of all recorded neurons ( grey ). Dashed line indicates chance level. Vertical lines mark the beginning of the rule-cue period, end of the rule-cue period and end of the Delay2 period. Full size image Single neurons encoded abstract rules Many single neurons varied their firing rates according to the abstract behavioural rule. 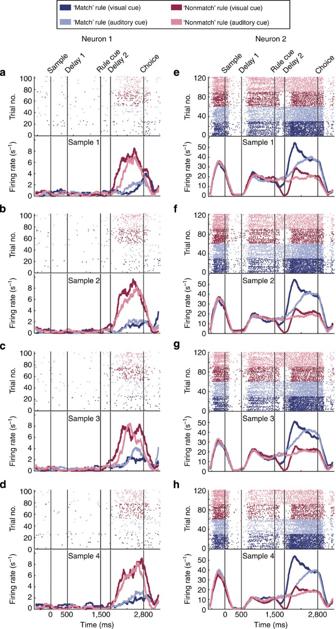Figure 6: Individual neurons in the NCL represent the abstract rules. (a–d) Example of a rule-selective neuron preferring the ‘nonmatch’ rule. This unit discriminated between the behavioural rules in the Delay2 period, irrespective of the sample stimulus or the modality of the cue.Top:Dot raster showing the neuron’s response in individual trials, ordered by the presented rule cue (each dot signifies one action potential).Bottom:peri-stimulus time histogram (PSTH), obtained by averaging the dot raster and smoothing with a 150 ms boxcar window. Vertical lines mark transitions between task periods, different panels show responses to different sample pictures. (e–h) Example neuron preferring the ‘match’ rule. This unit was strongly influenced by the sensory properties of the cue during the cue period and the first part of Delay2. At the end of the delay it only discriminated between the behavioural rule, irrespective of the cue modality. Figure 6a–d shows an example neuron that reliably discharged after rule-cue presentation whenever the ‘nonmatch’ rule was in effect, irrespective of whether it was instructed by a visual cue or an auditory cue. Other neurons showed the reversed preference and responded maximally to the ‘match’ rule ( Fig. 6e–h ). The neuron in Fig. 6e–h reflected the cue modality shortly after rule-cue onset but encoded only the abstract rule later in the Delay2 phase. Figure 6: Individual neurons in the NCL represent the abstract rules. ( a – d ) Example of a rule-selective neuron preferring the ‘nonmatch’ rule. This unit discriminated between the behavioural rules in the Delay2 period, irrespective of the sample stimulus or the modality of the cue. Top: Dot raster showing the neuron’s response in individual trials, ordered by the presented rule cue (each dot signifies one action potential). Bottom: peri-stimulus time histogram (PSTH), obtained by averaging the dot raster and smoothing with a 150 ms boxcar window. Vertical lines mark transitions between task periods, different panels show responses to different sample pictures. ( e – h ) Example neuron preferring the ‘match’ rule. This unit was strongly influenced by the sensory properties of the cue during the cue period and the first part of Delay2. At the end of the delay it only discriminated between the behavioural rule, irrespective of the cue modality. Full size image To determine whether single neurons encoded the different task parameters in the Delay2 period, we used a three-way analysis of variance (ANOVA) to examine each neuron’s discharge rates in a 600 ms window before test onset, with the factors ‘sample picture’, ‘cue modality’ and ‘behavioural rule’ ( P <0.01, n =336). Both neurons in Fig. 6 showed a significant main factor ‘rule’ and no other main factors or interactions. In total, 15% (50/336) of all neurons recorded from the NCL encoded only the abstract rule (ANOVA, main factor ‘rule’, no other main factors or interactions, P <0.01, Fig. 7a ). An additional 5% (18/336) of all neurons exhibited other main factors in addition to the behavioural rule (significant main factor ‘rule’ and other main factors, no interactions, Fig. 7a ). These 68 neurons (20%) will be referred to as ‘rule neurons’ and further analysed below. We did not consider neurons with a main factor ‘rule’ and interactions with other main factors because these cells would typically respond to only one of the two-rule cues and thus not represent the abstract behavioural rule. 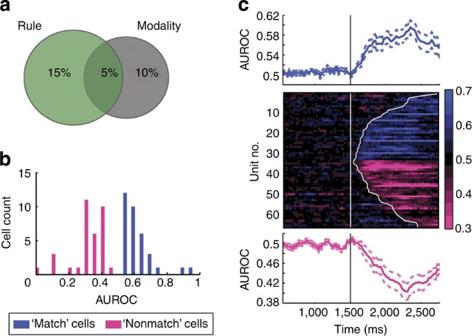Figure 7: Characterization of rule-selective neurons. (a) Results of an ANOVA with the factors ‘rule’, ‘cue modality’ and ‘sample picture’. Fifteen percent of NCL neurons encoded only the abstract behavioural rule, with an additional 5% exhibiting main factors of ‘rule’ and ‘modality’ (but no interaction between factors). (b) Quality of rule coding. Histogram of AUROC values of all rule neurons. By convention, values <0.5 represent neurons preferring the ‘nonmatch’ rule (pink), values >0.5 represent neurons preferring the ‘match’ rule (blue). There were equal numbers of neurons preferring each rule. (c) Time course of rule selectivity for all rule neurons. Neurons are sorted based on their rule preference and the latency of rule selectivity.Middle:AUROC values of each individual rule neuron throughout the Delay2 period. The white bar at 1,500 ms indicates the onset of the rule cue. The white line marks each neuron’s latency of rule discrimination.Top:average AUROC values of all neurons preferring the ‘match’ rule.Bottom:average AUROC values of all neurons preferring the ‘nonmatch’ rule. Dashed lines show s.e.m.,n=33 each. Figure 7: Characterization of rule-selective neurons. ( a ) Results of an ANOVA with the factors ‘rule’, ‘cue modality’ and ‘sample picture’. Fifteen percent of NCL neurons encoded only the abstract behavioural rule, with an additional 5% exhibiting main factors of ‘rule’ and ‘modality’ (but no interaction between factors). ( b ) Quality of rule coding. Histogram of AUROC values of all rule neurons. By convention, values <0.5 represent neurons preferring the ‘nonmatch’ rule ( pink ), values >0.5 represent neurons preferring the ‘match’ rule ( blue ). There were equal numbers of neurons preferring each rule. ( c ) Time course of rule selectivity for all rule neurons. Neurons are sorted based on their rule preference and the latency of rule selectivity. Middle: AUROC values of each individual rule neuron throughout the Delay2 period. The white bar at 1,500 ms indicates the onset of the rule cue. The white line marks each neuron’s latency of rule discrimination. Top: average AUROC values of all neurons preferring the ‘match’ rule. Bottom: average AUROC values of all neurons preferring the ‘nonmatch’ rule. Dashed lines show s.e.m., n =33 each. Full size image Table 1 shows that the most prevalent activity in the second half of the Delay2 period recorded from randomly selected NCL neurons represented the abstract rules (for proportions of neurons selectively tuned to the factors ‘sample picture’, ‘cue modality’, ‘behavioural rule’ and ‘target location’ in other task periods, see Table 2 ). Rule neurons encoded only the behavioural rule while abstracting over different sample pictures and different cues. Sensory factors could not account for differential responses to the rules in the Delay2 period because each rule was instructed using cues from two different sensory modalities. Motor preparation or reward expectation could also be excluded as the crow could not know whether the correct object would appear on the left or right side of the screen, and the expected reward was identical for all rules. Thus, the selective neuronal responses are a correlate of abstract encoding of the behavioural rule. We defined a rule neuron’s ‘preferred rule’ as the rule that elicited the highest discharge rate; we found equal numbers of rule neurons preferring the ‘match’ rule and the ‘nonmatch’ rule ( N =34 each, Fig. 7b ). Table 1 Percentage of cells selective in the Delay 2 period. Full size table Table 2 Neuronal selectivity in different task periods. Full size table We used a receiver operating characteristic (ROC) analysis to quantify how well the different rules could be discriminated based on the distribution of each rule neuron’s response rates in different trials. The area under the ROC curve (AUROC) is a measure of the separation of two distributions, with 0.5 indicating complete overlap, and both 0 and 1 indicating perfect separation. By convention (see Methods), neurons preferring the ‘match’ rule had AUROC values >0.5, and neurons preferring the ‘nonmatch’ rule had AUROC values <0.5 ( Fig. 7b ). The strength of rule coding measured by the ROC analysis was similar for neurons preferring the ‘match’ and ‘nonmatch’ rules (median AUROC=0.62, and median AUROC=0.36, respectively; P >0.05, Mann–Whitney U -test on rectified values between 0.5 and 1, n =34 each). To determine the latency of rule discrimination and to visualize the temporal evolution of rule selectivity for all rule neurons, we performed a sliding ROC analysis. Throughout the Delay2 period, an increasing number of rule neurons started discriminating the behavioural rules with a median latency of 260 ms after the onset of the rule cue ( Fig. 7c ). The average AUROC curves for the population of ‘match’-preferring and ‘nonmatch’-preferring neurons stayed consistently high ( Fig. 7c ), indicating that rule information was present in the population of rule neurons at each time point during the delay. Rule-coding neurons predicted the crows’ decision behaviour If the rule-coding neurons are relevant for the birds and predict their choice behaviour, their responses should differ in trials in which the birds made a mistake; that is, when they were instructed to use the ‘match’ rule, but they followed the ‘nonmatch’ rule instead, or vice versa . 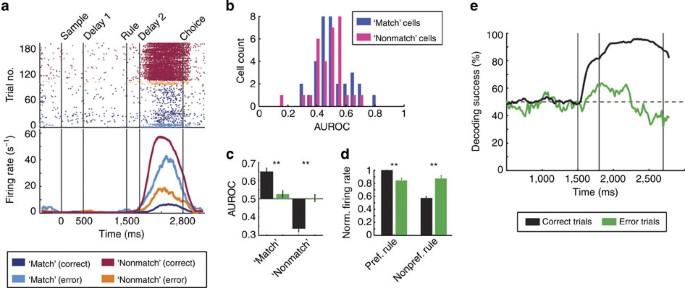Figure 8: Behavioural relevance of rule-selective neurons. (a) Responses of a ‘nonmatch’-preferring neuron during correct and error trials. In error trials, the firing rate for the ‘nonmatch’ rule was reduced, and the firing rate for the ‘match’ rule was increased. (b) Quality of rule coding in error trials. Histogram of AUROC values of all rule neurons in error trials. Pink bars represent neurons preferring the ‘nonmatch’ rule in correct trials, blue bars represent neurons preferring the ‘match’ rule in correct trials. (c) Average AUROC values of all rule neurons during correct and error trials. Error bars indicate s.e.m., asterisks indicate significant differences (**P<0.001, Wilcoxon-signed rank test,n=33 for ‘match’, 31 for ‘nonmatch’). (d) Firing rate of all rule neurons during correct and error trials, normalized so that each neuron’s response to its preferred rule in correct trials equals 1. Error bars indicate s.e.m., asterisks indicate significant differences (**P<0.001, Wilcoxon-signed rank test,n=68). (e) Decoding time course for correct and error trials, using a model trained on correct trials. Dashed line indicates chance level. Vertical lines mark the beginning of the rule-cue period, end of the rule cue period and end of the Delay2 period. Figure 8a shows an example neuron that responded vigorously to the ‘nonmatch’ rule in correct trials but only weakly to the ‘match’ rule. This neuron’s activity was inverted in error trials, now with a strong discharge whenever the crow made an error during the ‘match’ rule and followed the ‘nonmatch’ rule instead. To evaluate rule coding when the birds applied the wrong rule, we calculated AUROC values using discharge rates in error trials. In contrast to the identical neurons’ AUROC values for correct trials ( Fig. 7b ), discriminability was significantly reduced in error trials ( Fig. 8b ), for both the ‘match’ and ‘nonmatch’ rules ( P <0.001, Wilcoxon-signed rank test, n =33, 31, respectively; Fig. 8c ). The same was true if we artificially reduced the number of correct trials to match the number of error trials for each neuron ( P <0.01, Wilcoxon-signed rank test, n =33, 31, respectively). Moreover, we did not find a significant difference between the strength of rule coding in all correct trials and in correct trials with artificially reduced number of trials ( P >0.05, Wilcoxon-signed rank test, n =33, 31, respectively). Therefore, the reduced AUROC values in error trials are not a result of the reduced number of trials in error trials but rather stem from genuinely weaker rule selectivity in error trials. This resulted both from an increase in response rates to the non-preferred rule by 79.5%, as well as a decrease in activity to the preferred rule by 15.7% ( P <0.001, Wilcoxon-signed rank test, n =68; Fig. 8d ). In addition, the classifier decoding performance (when trained on correct trials) for error trials was dramatically reduced ( Fig. 8e ). Decoding performance at the end of the Delay2 phase tended to be lower than chance level—that is, error trials were more frequently classified as belonging to the opposite rule than to the instructed rule, mirroring the birds erroneous behavioural choice. Figure 8: Behavioural relevance of rule-selective neurons. ( a ) Responses of a ‘nonmatch’-preferring neuron during correct and error trials. In error trials, the firing rate for the ‘nonmatch’ rule was reduced, and the firing rate for the ‘match’ rule was increased. ( b ) Quality of rule coding in error trials. Histogram of AUROC values of all rule neurons in error trials. Pink bars represent neurons preferring the ‘nonmatch’ rule in correct trials, blue bars represent neurons preferring the ‘match’ rule in correct trials. ( c ) Average AUROC values of all rule neurons during correct and error trials. Error bars indicate s.e.m., asterisks indicate significant differences (** P <0.001, Wilcoxon-signed rank test, n =33 for ‘match’, 31 for ‘nonmatch’). ( d ) Firing rate of all rule neurons during correct and error trials, normalized so that each neuron’s response to its preferred rule in correct trials equals 1. Error bars indicate s.e.m., asterisks indicate significant differences (** P <0.001, Wilcoxon-signed rank test, n =68). ( e ) Decoding time course for correct and error trials, using a model trained on correct trials. Dashed line indicates chance level. Vertical lines mark the beginning of the rule-cue period, end of the rule cue period and end of the Delay2 period. Full size image Our findings demonstrate the cognitive flexibility of crows to go beyond fixed stimulus–response associations and to choose between strategies according to rules, a hallmark of executive function [14] , [38] , [39] . We report a neural correlate of rule-based executive control functions in the NCL, a higher association area and a proposed avian analogue of the PFC. Neurons in the NCL significantly varied their response rates according to the behavioural rule, while abstracting over different sample images and the sensory modality of the rule cues. In trials in which the birds made a mistake, rule coding was weaker or even reversed, suggesting that the activity of the recorded neurons was relevant to the birds’ behaviour on a trial-by-trial basis. The ability to guide behaviour by general rules rather than by relying on fixed stimulus–response associations constitutes a survival advantage; it allows animals to abstract from individual situations and flexibly act in a changing environment according to internal goals. Corvids have been shown to exhibit sophisticated executive control similar to primates [14] , [38] . For example, Eurasian jays flexibly switch their foraging tactics based on social context [7] , or scrub jays flexibly hide food according to their anticipated future needs [8] . Corvids readily abstract general principles from their tasks [11] . Here we show that crows acquire and follow abstract ‘match/nonmatch’ rules that they can apply to novel stimuli in a controlled conditioning approach. This recommends the crow as an excellent new model to study the neural basis of executive control in the absence of a six-layered neocortex. As expected for a telencephalic association brain area [32] , many neurons responded selectively to sensory, cognitive and/or motor task parameters that were relevant at that point in the trial (that is, identity of the sample stimulus or target location in the response phase). Of all the parameters investigated in the Delay2 period (working memory for the sample, sensory features of the rule cue and the rules themselves), the most prevalent single-unit activity recorded in NCL neurons represented the behavioural rules. We found that the discharge rates of 20% of randomly selected NCL neurons significantly discriminated the two rules (‘match’ or ‘nonmatch’), irrespective of the identity of the sample images. By instructing each rule with one of two-rule cues from different modalities, we could exclude purely sensory responses to the rule cues. We therefore consider the coding of rule-selective neurons to be highly abstract because it cannot be explained by sensory features and applies generally to all sample images. The activity of rule-selective neurons was behaviourally relevant and predicted the crows’ decision. When the crows chose the wrong item, the encoding of the rule by the population of rule neurons was weaker or even reversed in the preceding delay period. The weaker discrimination of the preferred and non-preferred rule was caused both by a decrease in activity to the preferred rule as well as an increase in activity to the non-preferred rule. Thus, the neurophysiological differences in error trials stemmed from the crows’ ‘confusion’ of the current rule, not from a general drop in activity caused by general attentional or motivational factors. This suggests that the birds relied on such rule-selective neurons when making a behavioural decision at the end of each trial. As we used a task with a similar level of difficulty and stimulus control as used in primate studies [30] , the activity of NCL neurons can be compared directly with neurons in the PFC of primates, the proposed functional analogue of the avian NCL [16] . Overall, a similar proportion of neurons (~20%) encoding the abstract rule seems to be present in both species. Moreover, the strength of rule selectivity is comparable in the crow’s NCL and in the PFC of monkeys [30] , [32] , [33] , [34] , [40] . Rule selectivity in the NCL emerged gradually with long latencies, mirroring rule-coding activity in the PFC of primates [32] . This temporal evolution of rule selectivity might reflect time-consuming cognitive processing of the cue and subsequent preparation of the appropriate response. Since rule-related activity has been found in multiple association areas of the primate endbrain [31] , [33] , rule-related activity might also be expected in other association areas of avian brains. The observed rule activity alone does not contain sufficient information to solve the task because it needs to be combined with working memory for the sample picture to make the correct choice. Moreover, this kind of abstract rule activity would not be strictly required to solve the task; for instance, an animal might encode each of the four cues separately. Therefore, the rule activity we observed represents a most abstract-processing step, whose existence is not evident from the task itself. The fact that both crows and monkeys form this abstract neuronal representation with different neural architectures but similar connectivity argues that having access to this highest level of abstraction constitutes a key computational principle for solving this and similar tasks. The prevalence of rule activity over other task parameters indicates that the abstraction of behavioural rules and principles may be an important function of both the corvid NCL and the primate PFC. This suggests that intelligent species of these distantly related animal groups found similar neurophysiological solutions through convergent evolution to master such cognitively demanding tasks. These findings add to the growing body of evidence for the functional analogy between NCL and PFC. Both areas share a large number of similarities in terms of connectivity, neurochemistry and function. Both NCL and PFC are multimodal association areas that operate at the top of the telencephalic-processing hierarchy [16] , [41] , ideally positioned to integrate sensory input and project to motor output [15] . Posterior movement-associated areas, such as the NCL, have been suggested to show activity related to movements and vocalizations [42] , again reflecting PFC function [43] , [44] . Moreover, like the PFC, the NCL is densely innervated by dopaminergic fibres from the midbrain [35] , [36] , [45] . Lesions in the NCL cause deficits in delayed alternation, visual working memory and reversal learning in pigeons [17] , [18] , [19] , mirroring equivalent dysfunctions after damage of the PFC [46] , [47] , [48] . Sustained delay activity is regarded to be a neuronal correlate of working memory in the PFC [49] , [50] . In pigeons, sustained delay activity was observed to encode working memory or reward prediction during delayed go/nogo tasks [20] and instructed forgetting tasks [21] , [51] , [52] . These similarities are surprising, considering the 300 million years of independent evolution and strikingly different neuroarchitecture of mammalian and avian brains. Our findings emphasize that birds, and corvids in particular, developed high-capacity endbrain circuitries without a six-layered neocortex independently of mammals via convergent evolution. Despite the differences in neuroarchitecture, birds and mammals share similarities on the level of neuronal circuits that enable highly sophisticated behaviour. For example, both birds and mammals share ascending sensory pathways that pass information through the thalamus to primary sensory areas [24] , then sensory association areas and finally multimodal association areas [16] . Therefore, higher association areas such as NCL or PFC are the key components of some of these shared neuronal circuits in birds and mammals. Understanding the differences and similarities in neuronal processing in these two functionally equivalent endbrain areas of different evolutionary origin will help to reveal the general principles and evolutionary constraints for the design of highly cognitive vertebrate brains. Subjects Two hand-raised, 1-year old male carrion crows ( Corvus corone corone ) weighing 530 and 570 g, obtained from the institute’s breeding facilities, were used in these experiments. The crows were 9 months old at the start of training. The birds were housed in social groups in spacious indoor aviaries [10] . The crows were maintained on a controlled feeding protocol during the sessions and earned food during and after the daily tests. The complete training procedure, including familiarization with the apparatus, training of the behavioural task, light barrier training and familiarization with recording procedures, lasted ~11 months. Slowly adjusting the behavioural protocol to the final rule-switching task required ~4 months of this time. Introduction of the light barrier and training the birds to keep their heads still required ~2 weeks of training. All procedures were carried out according to the University of Tübingen guidelines for animal experimentation and authorized by the Regierungspräsidium. Apparatus The crows were trained on a delayed rule-switching task in a fully controlled operant-conditioning chamber. They stood on a wooden perch attached by a leather jess and were placed in front of a touchscreen monitor (3 M Microtouch, 15′′, 60 Hz refresh rate) so that the monitor was within the beak’s reach. All visual stimuli were displayed on this touchscreen monitor. Reward for correct trials (birdseed pellets or mealworms ( Tenebrio molitor larvae)) was delivered by a custom-built automated feeder below the touchscreen. The CORTEX program (National Institute of Mental Health) was used for experimental control and behavioural data acquisition. An infrared light barrier in combination with a reflector attached to the bird’s head registered when the bird was positioned in front of the screen and facing it. Behavioural protocol The crows initiated a trial ( Fig. 1 ) by moving their heads into the light barrier whenever a go-stimulus (white square, 11 × 11 mm) was shown on the screen. The crows had to keep their heads still throughout the trial; if they moved their heads prior to the response period (as detected by the light barrier), the trial was aborted. After 200 ms, the go-stimulus turned off, followed by a 500 ms-presample period without any stimulus on the screen. Next, a sample stimulus was presented in the centre of the screen for 500 ms. Sample pictures were randomly chosen from a set of four photographs (20 × 20 mm) that was exchanged every day. After a first memory delay (Delay1; 1,000 ms), the rule (‘match’ or ‘nonmatch’) for any given trial was signified by a randomly chosen rule cue. The ‘match’-rule was indicated by either a blue circle (3 cm diameter) presented for 300 ms in the centre of the screen, or a frequency-modulated 1–4 kHz upward sweep (300 ms duration) played through a speaker. The screen remained black during auditory cue presentation. The ‘nonmatch’-rule was cued either by a red circle (3 cm diameter, 300 ms duration) or by a white-noise sound (300 ms duration). Thus, two distinct cues from different sensory modalities were used to indicate the same rules, whereas cues signifying different rules were from the same modality. This allowed to later separate the neural activity related to the physical properties of the cue from the rule that it signified. After the crows were instructed in the rule-cue phase, a second delay followed (Delay2; 1,000 ms). Finally, two images were presented for 1,200 ms side-by-side on the touchscreen in the choice period. During the choice period, the sample image as shown during the sample phase (‘match’) and one other image (‘nonmatch’) from the daily stimulus set (20 × 20 mm each) were presented 6.6 cm apart to the left and right of the centre. The location (left or right) of the ‘match’ and ‘nonmatch’ test image was randomized and balanced. The birds indicated their choices by pecking at the appropriate image on the touchscreen according to the rule in effect for each trial. A food item was dispensed by the automated feeder for each correct choice. Incorrect choices resulted in trial abortion, followed by a short time-out (3 s) prior to the start of the next trial. If no response occurred within 1,200 ms after choice onset, the trial was counted as an error. The four rule cues were presented pseudorandomly interleaved. All other relevant task parameters were balanced. Transfer test To test whether the crows grasped an abstract ‘match/nonmatch concept and were able to apply it to novel stimuli, we used transfer tests with pictures the birds had never seen before. For each crow, the transfer was tested in one session consisting of 420 trials with trial-unique sample items and nonmatch items. Every single sample image appeared only once during the transfer session, thus preventing any sample-specific learning. Apart from the trial-unique sample and choice stimuli, all other task parameters and contingencies were identical to the baseline protocol described under ‘Behavioral Protocol’. Baseline performance for comparison was measured in the days immediately before and after the transfer session. The results of the transfer tests are shown in Fig. 2b . Histology We applied immunohistochemical staining of brain sections to identify the target area of recordings, the NCL in the corvid telencephalon ( Fig. 3 ). For this purpose, two untrained crows were used. In pigeons, the NCL has been defined based on its dense dopaminergic innervation [35] . We used the density and distribution of tyrosine hydroxylase (TH)-immunoreactive fibres as a marker of dopaminergic innervation [36] characterizing the NCL [35] ( Fig. 3c ). As dopaminergic cells have to contain TH for the conversion of tyrosine into L-DOPA, all dopaminergic neurons must also be TH-positive. In addition, and similar to results in the pigeon brain, we found an abundance of so-called ‘baskets’ in the corvid NCL, which are characterized by TH-positive fibres coiled up like baskets around unlabelled perikarya ( Fig. 3d ). The Crows were anaesthetised with sodium pentobarbital (50 mg kg −1 ) and perfused with Ringer’s solution, followed by 4% paraformaldehyde in 0.1 M phosphate buffer at pH 7.4. The head was placed in a stereotaxic holder that was customized for crows in order to place markers to obtain stereotaxic coordinates of the brain sections. This stereotaxic holder allowed to hold the head in the standard orientation by placing the anterior fixation point (that is, beak bar position) 45° below the horizontal axis of the instrument, which is convention since the brain atlases by Karten and Hodos [53] . The brain was removed from the skull and blocked in sagittal or coronal planes. After post-fixation over night in 4% paraformaldehyde, the brain was transferred to a 20% sucrose in TBS (tris buffer) solution for 24 h, then a 30% sucrose in TBS solution for 48 h before sectioning. Cryostat sections (40 μm) cut in the coronal or sagittal planes were washed in TBS and treated for 5 min in TBS buffer (on microplate) containing H 2 O 2 . They were preincubated with 5% normal goat serum for 1 h at room temperature and then incubated with phosphate-buffered saline containing a rabbit antityrosine hydroxylase antibody (Anti-Tyrosine3-monooxygenase (TH), Catalogue No. AP08757PU-N, Rabbit Antibody IgG; Acris Antibodies, Herford, Germany; 1:500 Carrier) for 18 h at room temperature. After washing in TBS, sections were incubated with a biotinylated goat anti-rabbit IgG (affinity purified; Vector Laboratories, Burlingame, CA, USA; 1:1,000 in Carrier) for 1 h at room temperature and washed again in TBS. Finally, the sections were incubated with an avidin–biotin–peroxidase complex (VECTASTAIN Elite ABC Kit, Vector Laboratories; 1:1,000 in phosphate-buffered saline) for 1 h at room temperature. The peroxidase activity was visualized by incubating sections in 3,3′-diaminobenzidine. The nomenclature used in the present study is based on that of the Avian Brain Nomenclature Consortium [54] . A detailed histological study of the crow’s NCL is in preparation. Surgery and recordings All surgeries were performed while the animals were under general anaesthesia. The head was placed in the stereotaxic holder that was customized for crows with the anterior fixation point (that is, beak bar position) 45° below the horizontal axis of the instrument [53] . Using stereotaxic coordinates (centre of craniotomy: AP 5 mm; ML 13 mm), we chronically implanted two microdrives with four electrodes each, a connector for the headstage and a small headpost to hold the reflector for the light barrier. The crows received postoperative analgesics. We recorded from eight chronically implanted glass-coated tungsten microelectrodes (2 MΩ impedance, Alpha Omega LTD, Israel) on two custom-built microdrives in the left hemisphere. The electrodes targeted the NCL of the telencephalon. In a different crow implanted with the same stereotaxic coordinates, the location of the electrodes was histologically verified to lie in the NCL. A total of 132 neurons were recorded in bird D and 204 neurons in bird P. At the start of each session, the electrodes were advanced manually to obtain high-quality recordings. Each microdrive had a lift of ~5 mm, which was exploited to record from the NCL across different depths over a period of several weeks (43 recording sessions for bird D, 54 recording sessions for bird P). Neurons were not preselected for any involvement in the task. Signal amplification, filtering and digitizing of spike waveforms were accomplished using the Plexon system (Dallas, TX, USA). For each recording session, the birds were placed in the recording setup, a headstage containing an amplifier was plugged into the connector implanted on the bird’s head and connected to a second amplifier/filter and the Plexon MAP box outside the setup by a cable above and behind the bird’s head (all components by Plexon). Single-cell waveform separation was performed off-line (Plexon Systems). The analysis includes all neurons with a firing rate of at least 1 Hz during the entire trial. Each recording session lasted for ~500 correct trials in ~2 h. Explained variance analysis To quantify the factors affecting the firing rates of the entire population of recorded neurons, we calculated the variance explained by the different task variables (behavioural rule, cue modality and their interaction). The percent-explained variance ( ω 2 ) reflects how much of the variance in a neuron’s firing rates can be explained by the individual factors. The percent-explained variance for two factors was calculated using the MATLAB effect size measures toolbox [55] in a 300 ms-sliding window, advanced in steps of 20 ms. All statistical tests were carried out in MATLAB or R. Population-decoding analysis To investigate the quality of information about the cue modality and the behavioural rule provided by the entire population, we performed a population-decoding analysis based on a k -Nearest-Neighbor algorithm [37] using the MATLAB statistics toolbox with fivefold cross-validation. The k -Nearest-Neighbor algorithm is a simple classification method that classifies points based on actual examples in the training set and therefore contains no preassumptions about the underlying distribution of data points. Each point in the test set is assigned the same class as the majority vote of its k nearest neighbours in the training set ( Fig. 5b ). For the decoding of the behavioural rule, we classified individual trials as belonging to the ‘match’ or ‘nonmatch’ behavioural rule. For the decoding of cue modality, we classified individual trials as belonging to the visual or auditory cue modalities. Each trial is represented as one point in the n-dimensional feature space spanned by the firing rates of n neurons during this trial. Its neighbours are those training points with the smallest Euclidean distance to the test point in this n-dimensional feature space. A test point is assigned the same class as the majority vote of its k nearest neighbours. For example, if k =1, each trial would be classified as the same class as its neighbouring trial—that is, the trial with the smallest Euclidean distance in the space of firing rates of all neurons. We used k =31 neighbours; however, the relative performance for rules, cue modalities and correct versus error trials did not depend on the exact number of neighbours. Each unit with at least 80 trials for each rule and 80 trials for each cue modality was included in this analysis ( N =286). From all available trials, 80 trials for each classified condition were selected randomly and the trial timing was assigned randomly to create a population of pseudosimultaneously recorded neurons. This data set was then split up into five partitions, where four partitions were used as a training set and one partition was used as a test set (fivefold cross-validation). Cross-validation ensures that the test data are never used to train the model that they are tested on, thus preventing overfitting or an overestimation of the true classification power. Each test trial was assigned the same label as the majority vote of its 31 neighbouring trials in the training set with the smallest Euclidean distance in the 286-dimensional space of firing rates. This was repeated for all five partitions, so that each trial was part of the test set exactly once. We obtained a decoding time course by performing this analysis in a 100 ms window, advanced in steps of 20 ms. The entire procedure of selecting trials, assigning simultaneity, training and testing the model was repeated 100 times to account for differences in selecting the data. Selection of rule-selective neurons Neuronal activity (discharge rates) was analysed during the Delay2 period in a 600 ms window, starting 400 ms after rule-cue offset and lasting until the end of Delay2. A three-factor ANOVA with main factors ‘sample’ (four images), ‘rule cue’ (visual or auditory) and ‘rule’ (‘match’ or ‘nonmatch’) was used to determine whether the discharge rates of a neuron varied significantly with the identity of the sample stimulus, cue modality or the behavioural rule ( P <0.01). All neurons with a main effect of ‘rule’, but no interaction with other factors, were classified as ‘rule neurons’. The rule that elicited the largest discharge rate was defined as the preferred rule of a given cell. Analysis of selective neurons in other task periods Activity was analysed during different periods of interest throughout the trial (see data in Table 2 ). Firing rates during all additional task periods were calculated in 500 ms windows: for the sample period starting 100 ms after sample onset, for Delay1 period starting 100 ms after sample offset, for the cue period starting with onset of the rule cue and for the response period starting 500 ms before the bird’s response. For the sample period and Delay1 period, we calculated a Kruskal–Wallis one-way ANOVA in each window for the factor ‘sample picture’. For the rule-cue period and Delay2 period, a three-factor ANOVA with factors ‘sample picture’, ‘rule cue modality’ and ‘behavioural rule’ was applied. Finally, a four-factor ANOVA with factors ‘sample picture’, ‘rule cue modality’, ‘behavioural rule’ and ‘choice target location’ (left versus right target) was calculated in the response period. All ANOVAs were evaluated at P <0.01. ROC analysis We quantified the quality of rule encoding for each rule-selective unit using the ROC analysis derived from signal detection theory [56] . AUROC values were calculated based on the response rates in the same window as used for the ANOVA in the Delay2 period. Discharge rates for the ‘nonmatch’ rule were taken as reference distribution (‘noise’ distribution), whereas response rates to the ‘match’ rule constituted the test distribution (‘noise+signal’ distribution). For neurons that did not discriminate the rules and thus had completely overlapping distributions, the AUROC value was 0.5. Neurons preferring the ‘match’ rule showed an AUROC value >0.5, and neurons preferring the ‘nonmatch’ rule exhibited values <0.5. The magnitudes of AUROC values for neurons preferring the ‘match’ and ‘nonmatch’ rules were compared by first subtracting the AUROC values for the ‘nonmatch’ rule from 1, so that both distributions ranged from 0.5 to 1. In addition, a sliding ROC analysis was performed in a 100 ms window that was advanced in steps of 20 ms to determine the temporal evolution of the AUROC values throughout the Delay2 period. To test for significance, we used a permutation test to create a null distribution of AUROC values around 0.5 (by randomly assigning the labels ‘match’ and ‘nonmatch’ to different trials 1,000 times) for each neuron. A cell’s actual AUROC values were determined to be significantly different from 0.5 if they exceeded the lowest or highest 2.5th percentile of this null distribution ( P <0.05). The latency of rule selectivity was assigned as the first window of three consecutive windows with AUROC values that were significantly different from 0.5. The latency could not be determined for two-rule neurons; these cells are excluded from Fig. 7c . Error trial analysis We performed error trial analyses with the rule neurons ( N =68) selected using the ANOVA. Only rule neurons with at least three error trials for each rule were included in the ROC analyses of error trials ( N =64). Error ROC values were obtained by comparing the distribution for each cell’s preferred and non-preferred rules during error trials. Control ROC values for correct trials with matched number of trials were obtained by randomly selecting the same number of correct trials as available error trials for each neuron from the pool of all available correct trials. All rule neurons ( N =68) were included in the analysis of firing rates in error trials. Firing rates were normalized by dividing each neuron’s firing rates by its response to its preferred rule in correct trials. All rule neurons with a minimum of six error trials and 80 correct trials for each rule were used for the population-decoding analysis of error trials ( N =57). The classifier was trained on the cells’ firing rates in correct trials and then used to classify error trials. Therefore, error trials were classified according to the class of correct trials that they resembled most. How to cite this article: Veit, L. et al . Abstract rule neurons in the endbrain support intelligent behaviour in corvid songbirds. Nat. Commun. 4:2878 doi: 10.1038/ncomms3878 (2013).